Ginzburg–Landau-type theory of spin superconductivity Spin superconductivity is a recently proposed analogue of conventional charge superconductivity, in which spin currents flow without dissipation but charge currents do not. Here we derive a universal framework for describing the properties of a spin superconductor along similar lines to the Ginzburg–Landau equations that describe conventional superconductors, and show that the second of these Ginzburg–Landau-type equations is equivalent to a generalized London equation. Just as the GL equations enabled researchers to explore the behaviour of charge superconductors, our Ginzburg–Landau-type equations enable us to make a number of non-trivial predictions about the potential behaviour of putative spin superconductor. They enable us to calculate the super spin current in a spin superconductor under a uniform electric field or that induced by a thin conducting wire. Moreover, they allow us to predict the emergence of new phenomena, including the spin-current Josephson effect in which a time-independent magnetic field induces a time-dependent spin current. Superconductivity was discovered about a century ago [1] . It has attracted worldwide attention owing to its fascinating properties and many applications. It is still one of the central subjects in condensed matter physics. The mechanism of superconductivity can be understood by the Bardeen–Cooper–Schrieffer (BCS) theory [2] , which shows that electrons in the superconductor can form Cooper pairs and condense into the BCS ground state. Each Cooper pair contains electric charge 2 e , and usually is spin singlet. Recently, a new quantum state, named the spin superconductor, was proposed [3] , [4] . The spin superconductor is the counterpart of the charge superconductor. It is formed by condensed bosons in sufficiently low temperatures. The bosons are electrically neutral and their spins are non-zero. On one hand, the spin superconductor allows dissipationless flow of spin current and the spin resistance is zero. On the other hand, the charge current cannot flow through it and it is a charge insulator. Moreover, an electric Meissner effect against a spatial varying electric field exists in the spin superconductor [3] . The spin superconductivity may exist in spin-polarized triplet exciton systems of the graphene [3] , [4] , [5] , [6] , [7] , [8] , [9] , [10] , some three-dimension ferromagnetic materials, Bose–Einstein condensate of magnetic atoms, 3 He superfluidity and so on. Furthermore, the BCS-type theory, London-type equations and spin-current Josephson effect in the spin superconductor have also been presented [3] . In the history of superconductivity, another well-known theory, named the Ginzburg–Landau (GL) theory [11] , has also had an important role. The GL theory gives the phenomenological description of the superconductivity. In this Article, we derive the GL-type equations of the spin superconductor. Moreover, we show that the second GL-type equation is the generalized London-type equation, and analyse the characteristic parameters of the spin superconductor. Furthermore, we use the GL-type equations to calculate the super spin current in a spin superconductor under a uniform electric field and the super spin current where a thin charged wire is brought into the vicinity of a quasi two-dimensional (2D) spin superconductor. Finally, we use the GL-type equations to study the spin-current Josephson effect of the spin superconductor. We show the DC spin-current Josephson effect, the AC spin-current Josephson effect and the effect of an external electric field. The GL-type equations of spin superconductors To derive the GL-type equation, we should first write out the free energy of the system. For the spin superconductor under an external electric field E , the free energy can be represented as , where In equation (1), is the quasi-wave function of the spin superconductor. f s and f n are densities of free energy of the superconducting state and normal state, respectively. α ( T ) and are the low-order terms in the series expansion of the free energy f s , which are the same as the terms in the free energy of the charge superconductor [11] . The specific expressions of α ( T ) and β ( T ) can be obtained using the method proposed by Leggett [12] . Similar calculations manifest that they are also the same as the charge superconductor. can be seen as the kinetic energy and the spin–orbit coupling term, where m * is the effective mass of the carriers and α 0 is the coefficient of the spin–orbit coupling. The usual form of the spin–orbit coupling term is , where and . Here we consider the Hamiltonian being with , in which the first and second terms are the kinetic energy and the spin–orbit coupling, respectively. The third term ( E × s ) 2 is very small and is usually ignored. However, this term cannot be omitted in our derivation, because it contains the electric field E and its variation is not small. In fact, if we start with the Dirac equation of an electron in a potential ϕ and vector potential A , and take the non-relativistic limit, the canonical kinetic momentum can be written as [13] p canonical =− iħ ∇ + A + α 0 s × ∇ ϕ , thus H = ( p + α 0 s × ∇ ϕ ) 2 for the charge-neutral carrier. Similar with the vector potential A , the s × ∇ ϕ term has a role of a SU(2) gauge vector potential. In addition, if we start from the Hamiltonian H = ( p + α 0 s × ∇ ϕ ) 2 − m·B , and use the Hamilton canonical equations, we can get the correct equation of motion of a magnetic moment in the external electric field and magnetic field. In above expression, the field E has been written as − ∇ ϕ . This is reasonable because ∇ × E =0 is always tenable in our system [14] , [15] , [16] . The last term ε 0 ( ∇ ϕ ) 2 in equation (1) is the energy of the electric field. Note that the electric field E contains both the external field and the field induced by the super spin current. Next, we can use the variational method to obtain the GL-type equations. If we minimize the free energy with respect to the complex conjugate of the wave function, we get equation (2): In this derivation, we use the boundary condition: If we minimize the free energy with respect to the electric potential ϕ , we get equation (4): where ρ =− ε 0 ∇ 2 ϕ is the charge density. Equations (2) and (4) are the centre results of this paper. They are the first and second GL-type equations of the spin superconductor. This GL-type equations are universal to all spin superconductors and can also be used to study most of their properties and behaviours, including the electric Meissner effect, the spin-current Josephson effect, the proximity effect and their responses under an applied electromagnetic field. To see the physical meaning of equation (4) clearly, we make a simple transformation. We use the standard spin-current definition [15] , [17] , [18] , [19] with the velocity operator . Equation (4) is written as ρ =− ∇ ·( j s × α 0 s ). Here j s is the super spin current. As the spin is a vector, the spin current is a tensor product of the carrier current and the spin vector [15] , [17] , [18] , [19] . However, the direction of the spin is fixed in the spin superconductor; thus, we can use a vector j s , which describes the carrier current to represent the super spin current. The GL equations in equations (2) and (4) are time independent and we can obtain ∇ · j s =0 from them. It is the special case of the continuity equation when the system is time independent. As the usual spin current, the super spin current j s can generate an electric field E in space [14] , [15] , [16] , which is the same as that generated by the electric dipole moment. j s × α 0 s is the equivalent electric dipole moment P e . Next, ρ =− ∇ · P e can be seen as the equivalent charge induced by the spin current. Thus, the second GL-type equation describes the equivalent charge induced by the super spin current. This is different from the second GL equation of the charge superconductor, which describes the super current itself [11] . The relation between the GL-type and London-type equations By substituting into equation (5), we get Here, is the spin superfluid carrier density. Equation (6) can be seen as the generalized London-type equation. This is manifested as follows. If n s is independent of r , and take the curl of equation (6), we can get ∇ × j s = [( ∇ · E ) s −( s · ∇ ) E )]. In addition, the derivation of the second London-type equation in [3] does not consider the effect of electric charge in the system. Thus, we can take ∇ · E =0, then we obtain ∇ × j s = ( s · ∇ ) E . It is the same as the second London-type equation deduced in [3] . The characteristic lengths of the spin superconductor As we know, the charge superconductor has three characteristic parameters: the GL coherence length ξ , the penetration depth of the magnetic field λ and the GL parameter κ . In the following, we will analyse the characteristic parameters of the spin superconductor from the GL-type equations. First, if we set E =0, we can find that the GL-type equations of the spin superconductor are the same as the charge superconductor [20] when A =0. Therefore, the definition of the GL-type coherence length is also the same, that is ξ 2 ( T )= . Second, in the charge superconductor, the super current is j e ∝ A . It means that the first derivative of j e is proportional to the magnetic field B . Considering the Maxwell equation ∇ × B = μ 0 j e , we get ∇ 2 B ∝ B . From this equation, we can see that the magnetic field B decays exponentially from the surface to the interior. For the spin superconductor, however, the super spin current is j s ∝ E ; it is proportional to the electric field. As a result, the penetration depth λ is impossible to define, so is the GL-type parameter κ . The super spin current induced by a uniform electric field As an application of the GL-type equations, we use them to calculate the super spin current when a spin superconductor confronts a uniform electric field. When the field is sufficiently high, the spin superconductivity is destroyed. If we continuously decrease the field, at a certain field E = E c , spin superconductivity begins to appear. The E c is called the critical electric field. In the region where the field is very close to the critical field E c , the spin superconductivity is just beginning to appear; therefore, is very small. As a result, we can linearize the first GL-type equation [20] , [21] , [22] as: Suppose the surface of the spin superconductor lies in the xy plane and the uniform electric field is parallel to the surface, pointing to the y axis direction. The electric field can be written as E = E 0 e y , and we have . Here we have assumed that the direction of the spin s is fixed at z direction by the external field. By substituting into equation (7), we get The form of equation (8) is similar to the Schrödinger equation, and the left part can be regarded as . As , and are commutative with , the eigenfunction can be chosen as . The magnitudes of p x , p y and p z are determined by the boundary conditions and external conditions. We can choose the proper condition that makes p x = p y = p z =0, that is, we consider the case that the super spin current is zero when E =0. Under this case, we use to represent the wave function, which is uniform in the space. According to equation (5), we obtain . It should be noted that the super spin current j s is non-zero in the existence of the electric field E . The equivalent dipole moment is ; thus, the equivalent charge is Q =− ∇ · P e =0. Q =0 illustrates that the spin superconductor does not screen the electric field. This result is corresponding to the electric Meissner effect of the spin superconductor [3] , which says what the super spin current screens is the gradient of the electric field rather than the electric field itself. We can compare it with the case in the charge superconductor [20] . Suppose there is a uniform magnetic field parallel to the surface of the superconductor. The momentum p should be replaced by . The magnetic field B is the first-order differential of A ; therefore, if B is uniform, A is a linear function of r . By substituting it into the first GL-type equation of the charge superconductor, we get a potential energy that is a quadratic function of r . This equation is similar to the Schrödinger equation of the harmonic oscillator; thus, the solution is a local wave function. As a result, the super current is distributing near the surface. This super current can screen the magnetic field, producing the Meissner effect in the charge superconductor. In the spin superconductor, however, the momentum is changed to p − α 0 s × E . When the electric field is uniform, and by substituting it into the first GL-type equation, we get a constant potential. This potential cannot cause any non-trivial modification and the super spin current cannot be localized near the surface. In fact, the fundamental cause of this difference is that the electric charge is monopole but magnetic moment is dipole. It is the major asymmetry between electricity and magnetism. This cause the different Meissner effects for the charge superconductor and the spin superconductor. The super spin current induced by a thin charged wire Next, we calculate the super spin current when a quasi 2D spin superconductor confronts a field induced by a thin charged wire. As shown in Fig. 1a , a thin charged wire is on the top of a quasi 2D spin superconductor. The spin superconductor is a thin film and its thickness of the z direction is less than the GL-type coherent length ξ . Thus, the wave function is uniform in the z direction, which can be ignored. Furthermore, the thin film is infinite in the y direction, whereas the length in the x direction is finite. Suppose the charge density of the wire is ρ 0 , then the magnitude of the induced electric field is . As shown in Fig. 1 , the electric field can be written as . By substituting it into equation (7), and considering equations (4) and (5), we obtain the super spin current , the equivalent dipole moment P e ∝ j s × α 0 s ~ and the equivalent charge . The variation of the electric field induced by the super spin current along z direction, , is proportional to the equivalent charge . Note that , thus, the electric field induced by the super spin current cancels out . As a result, we can say that the super spin current screens the variation of the electric field. This conclusion, which is according to the electric Meissner effect of the spin superconductor, is also clearly clarified in Fig. 1b . It should be noted that the altitudes of the j s , Q and in Fig. 1b are meaningless, because we have ignored the coefficients. What Fig. 1b reflects is the tendency that the super spin current screens the variation of the electric field. We can also see that the flow direction of the super spin current in is opposite to that in x <0. In x =0, j s =0. 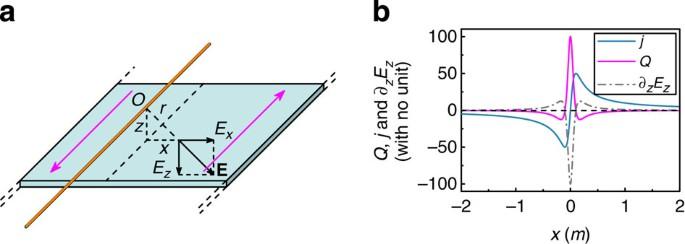Figure 1: The quasi 2D spin superconductor under a thin charged wire. (a) The schematic diagram for the device consisting of a thin charged wire and a thin film of spin superconductor. The red arrows describe the flow direction of the super spin current. (b) The variationof the electric field, the induced super spin currentjand the equivalent charge versusx. Figure 1: The quasi 2D spin superconductor under a thin charged wire. ( a ) The schematic diagram for the device consisting of a thin charged wire and a thin film of spin superconductor. The red arrows describe the flow direction of the super spin current. ( b ) The variation of the electric field, the induced super spin current j and the equivalent charge versus x . Full size image Spin-current Josephson effect of the spin superconductor We know that the Josephson effect is another highlight of the charge superconductor [23] . In the following, we use the GL-type equations to discuss the spin-current Josephson effect of the spin superconductor. The schematic diagram for the device is shown in Fig. 2 . We suppose that the magnetic fields, used to polarize the spins of electrons, are the same on both sides of the junction. When E =0, the GL-type equations of the spin superconductor are the same as the charge superconductor when A =0. Therefore, a spin superconductor has the same DC spin-current Josephson effect as a charge superconductor [23] . The super spin current is j = j 0 sin γ 0 , where γ 0 = γ 1 − γ 2 . j 0 is the Josephson critical super spin current, and γ 1 and γ 2 are phases of the spin superconductors on both sides of the Josephson junction. Next, consider the AC spin-current Josephson effect. As shown in Fig. 2a , the magnetic fields on both sides are different, B 1 = B 1 e z , B 2 = B 2 e z , B 1 ≠ B 2 . The super spin current flows from side 1 to side 2, and the change of phase is . Thus, we have . By substituting into the above equation, we get and . Therefore, the super spin current is j = j 0 sin( γ 0 + ω 0 t ), where . It can be seen that the super spin current is an alternating current. If the difference between the magnetic fields on both sides B 2 − B 1 is 0.01 T , we can estimate the frequency ω 0 , and its order of magnitude is 1 GHz. On the basis of this AC spin-current Josephson effect, we can very sensitively detect the spatial variance of the magnetic field by measuring the the frequency of the spin current. A difference of the magnetic fields, 2 × 10 −7 Gauss, can induce the spin current with its frequency around 1 Hz, which can be easily measured using the present technology. Next, we consider the effect of an external electric field shown in Fig. 2b . The uniform electric field is along the lateral direction of the Josephson junction and is written as E = E 0 e y . The phase is , where d is the width of the junction. Thus, the spin current is . It is changed by the sine rule according to the electric field. 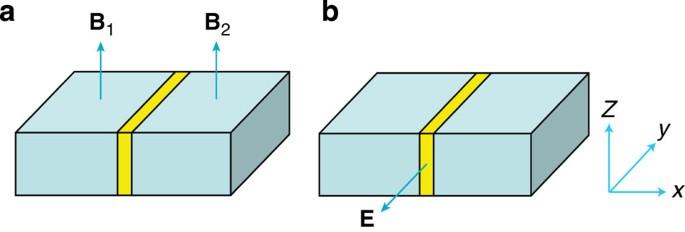Figure 2: The spin-current Josephson junction. (a) The schematic diagram for the device of Josephson junction (spin superconductor-insulator-spin superconductor junction). The magnetic fields imposed on both sides are unequalB1≠B2. (b) The schematic diagram for the device showing the effect of electric field on the spin-current Josephson effect. Figure 2: The spin-current Josephson junction. ( a ) The schematic diagram for the device of Josephson junction (spin superconductor-insulator-spin superconductor junction). The magnetic fields imposed on both sides are unequal B 1 ≠ B 2 . ( b ) The schematic diagram for the device showing the effect of electric field on the spin-current Josephson effect. Full size image In conclusion, we have derived the GL-type equations of the spin superconductor. We show that the second GL-type equation is the generalized London-type equation. In addition, we analyse some characteristic parameters of the spin superconductor by using the GL-type equations. Moreover, as the applications of the GL-type equations, we use them to calculate the super spin current in a spin superconductor under a uniform electric field and the super spin current where a thin charged wire is brought into the vicinity of a quasi 2D spin superconductor. Our result verifies the electric Meissner effect of the spin superconductor. We also discuss the spin-current Josephson effect of the spin superconductor from the GL-type equations, including the DC spin-current Josephson effect, the AC spin-current Josephson effect and the effect of an external electric field. To see the differences between the charge superconductor and the spin superconductor clearly, we summarize them in Table 1 . Table 1 The comparison of the charge and spin superconductors. Full size table The derivation of the GL-type equations At first, we minimize the free energy shown in equation (1) with respect to the complex conjugate of the wave function . For the second term of equation (1), we have For the third term of equation (1), we have For the fourth term, we get Note that and considering equations (9), (10), (11) and (12) together, we can obtain and Equation (13) is the first GL-type equation of the spin superconductor. Equation (14) is the boundary condition for the first GL-type equation, where the subscript n denotes the component perpendicular to the surface. On one hand, the boundary equation (14) can be viewed as the demand of the variational principle. The similar demand was adopted in the original paper written by Ginzburg and Landau [11] . On the other hand, the physical reason for choosing this boundary condition will be discussed shortly. If the wave function satisfies equation (13), it is easily shown that the super spin current is source free [24] , [25] , that is, ∇ · j s =0. In addition, if the wave function satisfy the equation (14) together, the spin superconductor sustains no net force. Next, we minimize the free energy with respect to the electric potential ϕ . For the fourth term of equation (1), we have For the fifth term of equation (1), we get Note that the total electric filed contains the external field and the field induced by the super spin current. The external field is fixed; thus, its result of variation is zero. We only need to minimize the free energy with respect to the field induced by the super spin current. Considerequations (15) and (16) together, we can obtain equation (17): where ρ =− ε 0 ∇ 2 ϕ . Equation (17) is the second GL-type equation of the spin superconductor. Solution of the super spin current under a thin charged wire By substituting the electric field into equation (7), we get The left part of equation (18) can be regarded as and is commutative with . Therefore, the eigenfunction can be chosen as . By substituting it into equation (18) and taking p y =0 (the value of p y is zero when we choose the external condition of the total super spin current being zero), we get By multiplying equation (19) by φ * and subtracting the product between the complex conjugate of equation (19) and φ , we have . By considering the boundary condition , we get . Therefore, at any point. It is easy to get, from the second GL-type equation, j x =0 and . Therefore, we have , the equivalent dipole moment , and the equivalent charge . How to cite this article: Bao, Z.-q. et al. Ginzburg–Landau-type theory of spin superconductivity. Nat. Commun. 4:2951 doi: 10.1038/ncomms3951 (2013).